Inhibition of endothelial ERK signalling by Smad1/5 is essential for haematopoietic stem cell emergence The earliest HSCs are derived from haemogenic endothelium via endothelial-to-haematopoietic transition during vertebrate embryogenesis; however, the underlying mechanism is largely unclear. Here we show that interplay of Smad1/5 and ERK signalling is essential for haemogenic endothelium-based HSC emergence. Smad1/5 directly inhibits erk expression through recruiting HDAC1 to and inducing de-acetylation of the erk promoter in endothelial cells. Over-activated ERK signalling conferred by inhibition of Smad1/5 promotes the arterial endothelial cell fate and constitutively strengthens the tight junction between endothelial cells, thereby repressing the specification of haemogenic endothelium and the following endothelial-to-haematopoietic transition process. These findings provide new insights into the in vitro generation of transplantable HSCs for potential clinical applications. Haematopoietic stem cells (HSCs), which are capable of differentiating into all blood lineages throughout the lifetime, are generated via a process named endothelial-to-haematopoietic transition (EHT) during embryogenesis in vertebrates [1] , [2] , [3] . During EHT, a subset of endothelial cells in the aortic floor develop into haemogenic endothelial cells regulated by a combination of transcription factors and signalling pathways such as Runx1 (refs 1 , 4 ), ETS factors [5] , [6] and Hedgehog-Notch-Scl pathway [7] . These cells then bend and turn round under the regulation of gfi1 and gfi1b [8] . Consequently, they lose their endothelial identity and the surrounding tight junction and egress into the subaortic space in zebrafish or into the intra-aortic space in avian, Xenopus and mouse during embryogenesis [9] . F2r-RhoA/ROCK pathway inhibits this process through strengthening the tight junction [10] . In vitro , embryonic stem cells (ESCs) and induced pluripotent stem cell (iPSC)-derived haematopoietic stem/progenitor cells (HSPCs) make it feasible to investigate the molecular mechanisms underlying embryonic haematopoiesis. During ESC or iPSC differentiation into haematopoietic cells, different culture conditions have been optimized to promote haematopoietic cell production. Signalling pathways like Notch-Dll4 (ref. 11 ), VEGF and FGF, TGFβ (ref. 12 ) and BMP4 (ref. 13 ) have been reported to play important roles during in vitro haematopoietic differentiation process. Recapitulation of embryonic signalling events in vitro may help us to obtain unlimited supply of functional HSCs from pluripotent stem cells (ESCs, iPSCs) or even from different types of somatic cells (via transdifferentiation), which holds a great promise for regenerative medicine. BMPs, especially BMP4, can induce the formation of mesoderm and haematopoietic progenitor cells both in vivo and in vitro . BMP4 was implicated to act as a haematopoietic growth factor in Xenopus [14] . Using a dominant-negative zebrafish mutant, Wilkinson et al. [15] found that BMP signalling is required for the initiation and maintenance of definitive HSCs. Smad1 and Smad5, the key mediators of BMP signalling pathway, are involved in the regulation of haematopoiesis. In zebrafish, loss of either smad1 or smad5 affects the generation of definitive haematopoietic progenitors [16] . Nonetheless, the underlying molecular mechanism of Smads in definitive haematopoiesis remains to be elucidated. In mice, Smad1 transactivated the Runx1 transcription, while Smad6 inhibited the Runx1 transcription in conjunction with Smurf1 (ref. 17 ). Interestingly, recent studies revealed that Smad1 also transiently restricts the early expansion of haematopoietic progenitors, partially due to the repression of GATA1 transcription [18] . These data suggest that Smads might directly regulate expression of certain master regulators of haematopoietic lineages at the transcriptional level. The molecular mechanisms underlying the VEGF/FGF-induced ERK regulation of HSC are not very clear. Evidence available suggests that the VEGF regulation of HSC during development is primarily mediated by its early role in artery–vein specification [19] . The artery–vein determination is achieved mainly by antagonizing phosphatidylinositol-3 kinase (PI3K) and MAP kinase/ERK signalling pathways, which are the two signalling branches downstream of VEGF. Using different inhibitors of PI3K/AKT pathway and ERK pathway, Hong et al. [20] , [21] demonstrated that stimulation of ERK signalling promotes the artery specification, while such an effect of ERK can be inhibited by PI3K, and vice versa . In the artery, VEGF receptor 2, Flk1(Kdrl), transmits the signals to the downstream PLCγ/ERK branch and thus determines the arterial fate, while in the vein, VEGF receptor 3, Flt4, transmits the signals to the PI3K/AKT branch to determine the venous fate [20] . Previous studies showed that phosphorylated ERK was prevalent in the dorsal aorta at E9-9.5, then decreased in the established vessels, which is only detectable in the most nascent blood vessels in zebrafish and mouse embryos [20] , [22] . However, the molecular mechanisms of ERK action and transcriptional regulation of ERK expression in HSC fate determination and lineage differentiation have not been explored yet. Although these signalling pathways have been demonstrated to play pivotal roles during definitive haematopoiesis, several fundamental questions remain unanswered. For example, which biological process of HSC development is regulated by BMP and ERK signalling, respectively? How do they interact with each other to ensure a proper developmental sequence during HSC emergence in a stepwise manner? Here we show that persistently activated ERK in endothelial cells after artery–vein establishment promotes the arterial endothelial cell fate and strengthens the tight junction between endothelial cells, then repressing the specification of haemogenic endothelium and the following EHT process by which the earliest HSCs are derived. Therefore, after artery–vein specification, endothelial ERK signalling is no longer required and must be attenuated. We further demonstrate that BMP–Smad1/5 pathway can directly inhibit erk expression through recruiting HDAC1 to erk promoter. Our studies suggest that the cross-talk between BMP and ERK pathways maintains a favourable condition required for the HSC emergence in vertebrates. Smad1/5 is continuously required for the HSC initiation As an important morphogen, BMP signalling pathway is essential for early development in zebrafish. To avoid the early defects, a transgenic line (tBR) with heatshock-inducible dominant-negative bmpr1 and specific inhibitors were used at various stages after gastrulation. Whole-mount in situ hybridization (WISH) showed that in tBR embryos heat-shocked at 10 hpf (bud stage) or embryos treated with BMP inhibitor dorsomorphin (DM) [23] from 10 hpf, the expression of HSC markers runx1 at 24 hpf and cmyb at 36 hpf was decreased ( Supplementary Fig. 1a ), suggesting that after gastrulation stages, BMP signalling is still required for HSC specification. To further pinpoint the timing of BMP action precisely, more specific inhibitors (DMH1 and LDN193189) [24] were used at different stages. Our result showed that the expression of runx1 and cmyb was decreased in embryos treated with DMH1 and LDN193189, at 14, 20, 24 or 30 hpf ( Supplementary Fig. 1b ). Such observation was also recapitulated in Tg( kdrl :mCherry/ cmyb :GFP) double-transgenic lines, in which the kdrl + cmyb + cells were indicated as haemogenic endothelial cells [3] . The number of yellow ( kdrl + cmyb + ) cells was decreased in the embryos treated at 14, 24 or 30 hpf ( Supplementary Fig. 1c ). Together, these results suggested that the BMP signalling pathway is required for the initiation of HSCs or the EHT process at later stages (24 hpf and afterwards, that is, after gastrulation). To further explore the role of BMP signalling pathway in haematopoiesis, smad1 and smad5 morpholinos (MOs) [16] were employed. To avoid the early requirement during gastrulation at high concentration, low dose of smad1 or smad5 MOs were injected into embryos so that the embryos could develop relatively normally during and after gastrulation. Expression of runx1 and cmyb was remarkably reduced in smad1 and smad5 morphants ( Supplementary Fig. 1d ). To validate the WISH results, the same dose of smad1 or smad5 MOs was injected into Tg( kdrl :mCherry/ cmyb :GFP) double-transgenic embryos at the one-cell stage. Consistently, our results indicated that the number of kdrl + cmyb + cells was decreased at 36 hpf in smad1 and smad5 morphants ( Supplementary Fig. 1e ). Taken together, these data show that BMP–Smad1/5 pathway is essential for the haemogenic endothelial cell formation and HSC initiation. ERK is dynamically required for the HSC initiation MAPK/ERK signalling acts downstream of both FGF and VEGF pathways and is important for the artery–vein specification [21] . To determine whether FGF- or VEGF-induced ERK signalling is essential for definitive haematopoiesis, a transgenic line (dnFGF) with heatshock-inducible dominant-negative fgfr1 (ref. 25 ) and specific inhibitors for FGF (SU5402), VEGF (SU5416) [26] and MEK (PD98059) [20] were used to treat the embryos after gastrulation. The efficiency of these inhibitors in zebrafish embryos was validated by western blotting ( Supplementary Fig. 2a ). Interestingly, WISH showed that in the embryos treated with chemical inhibitors from bud stage (10 hpf), the expression of runx1 and cmyb was decreased ( Fig. 1a ), suggesting that FGF or VEGF signalling is required for definitive HSCs after gastrulation. 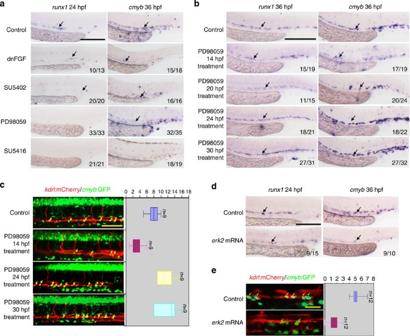Figure 1: ERK signalling pathway is required before artery-vein specification but not thereafter for the HSC initiation. (a) The expression ofrunx1at 24 hpf (left panels) andcmybat 36 hpf (right panels) was decreased in the dnFGF embryos heat-shocked at 10 hpf and embryos treated with FGF inhibitor SU5402, MEK inhibitor PD98059 or VEGF inhibitor SU5416 from 10 hpf (scale bar, 250 μm). (b) The expression ofrunx1at 36 hpf (left panels) andcmybat 36 hpf (right panels) was decreased in the embryos treated with PD98059 from 14 and 20 hpf, but increased in the embryos treated from 24 and 30 hpf (scale bar, 250 μm). (c) Confocal microscopy of Tg(kdrl:mCherry/cmyb:GFP) transgenic line at 36 hpf in control and embryos treated with PD98059 from 14 hpf, 24 hpf and 30 hpf, respectively. The yellow arrows mark the haemogenic endothelial cells (scale bar, 100 μm). The right panel showed the statistics ofkdrl+cmyb+cell numbers in the trunk region (mean±s.d.,n=9). (d) The expression ofrunx1at 24 hpf (left panels) andcmybat 36 hpf (right panels) was decreased inerk2mRNA-injected embryos (scale bar, 250 μm). (e) Confocal microscopy of Tg(kdrl:mCherry/cmyb:GFP) transgenic line at 36 hpf in control anderk2mRNA-injected embryos. The yellow arrows mark the haemogenic endothelial cells (scale bar, 50 μm). The right panel showed the statistics ofkdrl+cmyb+cell numbers in the trunk region (mean±s.d.,n=12). Figure 1: ERK signalling pathway is required before artery-vein specification but not thereafter for the HSC initiation. ( a ) The expression of runx1 at 24 hpf (left panels) and cmyb at 36 hpf (right panels) was decreased in the dnFGF embryos heat-shocked at 10 hpf and embryos treated with FGF inhibitor SU5402, MEK inhibitor PD98059 or VEGF inhibitor SU5416 from 10 hpf (scale bar, 250 μm). ( b ) The expression of runx1 at 36 hpf (left panels) and cmyb at 36 hpf (right panels) was decreased in the embryos treated with PD98059 from 14 and 20 hpf, but increased in the embryos treated from 24 and 30 hpf (scale bar, 250 μm). ( c ) Confocal microscopy of Tg( kdrl: mCherry/ cmyb :GFP) transgenic line at 36 hpf in control and embryos treated with PD98059 from 14 hpf, 24 hpf and 30 hpf, respectively. The yellow arrows mark the haemogenic endothelial cells (scale bar, 100 μm). The right panel showed the statistics of kdrl + cmyb + cell numbers in the trunk region (mean±s.d., n =9). ( d ) The expression of runx1 at 24 hpf (left panels) and cmyb at 36 hpf (right panels) was decreased in erk2 mRNA-injected embryos (scale bar, 250 μm). ( e ) Confocal microscopy of Tg( kdrl: mCherry/ cmyb :GFP) transgenic line at 36 hpf in control and erk2 mRNA-injected embryos. The yellow arrows mark the haemogenic endothelial cells (scale bar, 50 μm). The right panel showed the statistics of kdrl + cmyb + cell numbers in the trunk region (mean±s.d., n =12). Full size image As the common downstream effector, ERK plays pivotal roles in these signalling pathways. However, the exact role of ERK in HSC development was still controversial [5] , [27] . To clarify this, we first identified the timing of ERK action on HSC emergence. The time-course assay of erk1 and erk2 expression was performed. The transverse sections post WISH showed that the expression of erk1 and erk2 in endothelial cells was gradually decreased from 20–48 hpf ( Supplementary Fig. 2b ). Consistent results were also achieved by qPCR and western blotting analyses ( Supplementary Fig. 2c,d ). Then PD98059 was used at various developmental stages to inhibit ERK signalling. The results showed that the expression of runx1 and cmyb was decreased in the embryos treated before artery-vein specification (14 and 20 hpf, Fig. 1b ), but increased in the embryos treated at the stage between artery-vein specification and EHT process (24 and 30 hpf, Fig. 1b ). Moreover, in Tg( kdrl :mCherry/ cmyb :GFP) double-transgenic embryos treated at various stages, the number of kdrl + cmyb + haemogenic endothelial cells [3] was decreased in those treated at 14 hpf but increased in those treated at 24 or 30 hpf ( Fig. 1c ). These data together indicated that before artery-vein specification, ERK signalling is required for HSC emergence; while conversely, after artery-vein specification, it plays an inhibitory role on HSC development. Second, to identify the proper dose of ERK function in HSC initiation, we injected different doses of erk2 mRNA into the embryos at the one-cell stage. WISH showed that low dose of erk2 mRNA (<100 pg per embryo) increased the expression of HSC marker runx1 at 24 hpf and cmyb at 36 hpf ( Supplementary Fig. 2e ); however, when the dose was >150 pg per embryo, the expression of runx1 and cmyb was decreased ( Supplementary Fig. 2e ). In line with this observation, western blotting results confirmed that, while the increase of pERK level was evident after erk2 overexpression, the Runx1 expression was increased at low concentrations of erk2 mRNA but decreased at high concentration ( Supplementary Fig. 2f ). To further study the inhibitory role of ERK during haematopoiesis, erk2 mRNA with the dose of 200 pg per embryo was used in the following experiment. The results showed that, in erk2 -overexpressed embryos, the expression of runx1 at 24 hpf and cmyb at 36 hpf was decreased ( Fig. 1d ). Similarly, the number of kdrl + cmyb + cells was decreased at 36 hpf in these erk2 -overexpressed embryos ( Fig. 1e ). Taken together, these results suggested that ERK regulation of HSC emergence is biphasic: initially ERK plays an essential role in artery-vein specification; but after the establishment of artery-vein, ERK is not required for and even inhibits HSC emergence. Smad1/5 inhibits erk1 an d erk2 transcription BMP signalling has been reported to be able to inhibit activated ERK in certain cell types [28] , [29] . Therefore, we asked whether and how ERK signalling was turned down by the BMP–Smad1/5 pathway after artery-vein specification. Knockdown of smad1 or smad5 leads to similar HSC defects as overexpression of erk2 during HSC development ( Supplementary Fig. 1d,e , compared with Fig. 1d,e ), suggesting a possible negative relationship between BMP and ERK signalling. The transverse sections post WISH showed that the expression of erk1 and erk2 , especially in the endothelial cells was increased in smad1 and smad5 morphants ( Fig. 2a ). Quantitative RT–PCR (qPCR) confirmed the WISH results ( Fig. 2b ). Consistently, western blotting showed increased expression of total ERK and increased pERK, compared with control ( Fig. 2c ). Furthermore, the upregulation of ERK expression in smad1 and smad5 morphants was dose-dependent ( Supplementary Fig. 3a ). In addition, transgenic lines with expression of dominant-negative bmpr1 (tBR) and constitutively active bmpr1b (caBMP) were used to validate this inhibition. Results were consistent with the knockdown and overexpression of smad1/5 , respectively ( Fig. 2d ). In order to determine whether Smad1/5 directly inhibits ERK expression, smad1 and smad5 mis-match mRNAs [16] were injected to the embryos at the one-cell stage. It was found that the protein and RNA levels of ERK were decreased in these injected embryos in a dose-dependent manner ( Supplementary Fig. 3b,c ). To further confirm that the Smad1/5 inhibition of ERK occurs at the transcriptional level, specific inhibitors of VEGF (SU5416), FGF (SU5402) and MEK (PD98059) pathways were used to treat the smad1 or smad5 morphants. All of these inhibitors reduced the phosphorylation but not the expression of total ERK ( Supplementary Fig. 1a ). Western blotting showed that total ERK level remained upregulated, while the pERK level was attenuated by treatment with the inhibitors ( Fig. 2e,f ). Consistently, the qPCR results showed that the increased expression of both erk1 and erk2 was retained in smad1 or smad5 morphants treated with the inhibitors ( Fig. 2g,h ). Taken together, these results suggest that Smad1 or Smad5 inhibits ERK transcription. 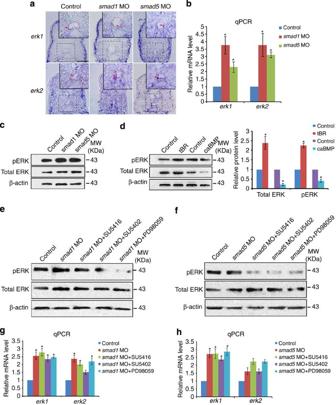Figure 2: Smad1/5 negatively regulates ERK transcription. (a) Transverse sectioning post WISH showed that the expression oferk1anderk2in the endothelial cells (red arrows in the black square) was increased in embryos injected withsmad1MO orsmad5MO. The red dotted lines mark the dorsal aorta (scale bar, 100 μm). (b) Quantitative RT–PCR analysis oferk1anderk2expression in the dissected trunk region of embryos injected with control MO,smad1MO andsmad5MO at 24 hpf (mean±s.d.,n=3,*P<0.05, Student’st-test). (c) Western blot showed that levels of both pERK and total ERK proteins were increased at 24 hpf in embryos injected withsmad1MO orsmad5MO. (d) Western blot showed that both pERK and total ERK levels were increased in tBR embryos but decreased in caBMP embryos. Quantification of the western result by using Quantity one software was presented in the right panel (mean±s.d.,n=3,*P<0.05, Student’st-test). (e,f) Western blot showed that the increase of pERK level but not the increase of total ERK level in embryos injected withsmad1MO (e) orsmad5MO (f) was inhibited by the treatment with SU5416, SU5402 or PD98059 from 10–24 hpf. (g,h) Quantitative RT–PCR analysis showed that the increased expression oferk1anderk2in embryos injected withsmad1MO (g) orsmad5MO (h) was not rescued by treatment with SU5416, SU5402 or PD98059 from 10–24 hpf (mean±s.d.,n=3,*P<0.05, Student’st-test). Figure 2: Smad1/5 negatively regulates ERK transcription. ( a ) Transverse sectioning post WISH showed that the expression of erk1 and erk2 in the endothelial cells (red arrows in the black square) was increased in embryos injected with smad1 MO or smad5 MO. The red dotted lines mark the dorsal aorta (scale bar, 100 μm). ( b ) Quantitative RT–PCR analysis of erk1 and erk2 expression in the dissected trunk region of embryos injected with control MO, smad1 MO and smad5 MO at 24 hpf (mean±s.d., n =3, *P <0.05, Student’s t -test). ( c ) Western blot showed that levels of both pERK and total ERK proteins were increased at 24 hpf in embryos injected with smad1 MO or smad5 MO. ( d ) Western blot showed that both pERK and total ERK levels were increased in tBR embryos but decreased in caBMP embryos. Quantification of the western result by using Quantity one software was presented in the right panel (mean±s.d., n =3, *P <0.05, Student’s t -test). ( e , f ) Western blot showed that the increase of pERK level but not the increase of total ERK level in embryos injected with smad1 MO ( e ) or smad5 MO ( f ) was inhibited by the treatment with SU5416, SU5402 or PD98059 from 10–24 hpf. ( g , h ) Quantitative RT–PCR analysis showed that the increased expression of erk1 and erk2 in embryos injected with smad1 MO ( g ) or smad5 MO ( h ) was not rescued by treatment with SU5416, SU5402 or PD98059 from 10–24 hpf (mean±s.d., n =3, *P <0.05, Student’s t -test). Full size image Smad1/5 recruits HDAC1 to regulate erk1/2 transcription Smad1 and Smad5 function as transcriptional factors in BMP signalling pathway [30] . Smads can recruit HDACs and other co-repressors onto the promoter of the target genes to inhibit their transcription [30] . In order to find out whether HDACs can mediate the Smad1/5 inhibition of ERK transcription during HSC development, we first used HDAC inhibitors trichostatin A and valproic acid [31] to treat zebrafish embryos at bud stage. Since HDAC1 was essential for HSC development [32] , we also performed hdac1 MO injection at the one-cell stage. The WISH results showed that the gene expression of HSC was decreased in the embryos with trichostatin A and valproic acid treatment or hdac1 knockdown, which was similar to those observed in smad1 or smad5 morphants ( Fig. 3a ). Then qPCR and western blotting experiments were performed to examine the expression of ERK at RNA and protein level. ERK expression was markedly increased in the HDAC inhibitor-treated or hdac1 knockdown embryos, compared with the control group ( Fig. 3b,c ). Then, we asked whether HDAC1 was involved in Smad1/5-induced ERK inhibition. To test this possibility, smad1 or smad5 mRNA was co-injected with hdac1 MO. As expected, with the deficient hdac1 expression, the inhibition of erk1 and erk2 caused by smad1 or smad5 overexpression was alleviated ( Supplementary Fig. 4a ). Western blotting also indicated that co-injection of hdac1 MO restored the decreased level of total ERK and pERK in smad1 or smad5 mRNA-injected embryos ( Supplementary Fig. 4b ). Taken together, these data indicate that HDAC1 mediates the Smad1/5 inhibition of ERK expression. 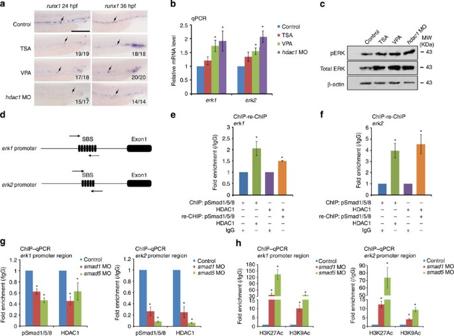Figure 3: HDAC1 is recruited by Smad1/5 to regulate histone acetylation on theerkpromoter. (a) The expression ofrunx1at 24 hpf (left panels) andrunx1at 36 hpf (right panels) was decreased in the embryos treated with trichostatin A or valproic acid (VPA) and embryos injected withhdac1MO (scale bar, 250 μm). (b) Quantitative RT–PCR analysis oferk1anderk2expression in the dissected trunk region of the embryos treated with TSA or VPA and embryos injected withhdac1MO at 24 hpf (mean±s.d.,n=3,*P<0.05, Student’st-test). (c) Western blot showed that both pERK and total ERK protein levels were remarkably increased in the embryos treated with TSA or VPA and embryos injected withhdac1MO at 24 hpf. (d) The diagram showed the Smad-binding sites in theerk1anderk2promoter region. The pair of arrows showed the primers designed for the ChIP assay. (e,f) ChIP-re-ChIP assay was performed for theerk1(e) anderk2(f) promoter region. Chromatin was precipitated with anti-pSmad1/5/8 or anti-HDAC1 antibody, and then re-precipitated with anti-HDAC1 or anti-pSmad1/5/8 antibody, respectively. Non-specific rabbit IgG was used as negative control (mean±s.d.,n=3,*P<0.05, Student’st-test). (g) ChIP assay was performed for theerk1(left) anderk2(right) promoter region in control embryos andsmad1/5morphants. DNA was immunoprecipitated with antibody against pSmad1/5/8 or HDAC1. The pSmad1/5/8 and HDAC1 enrichment was decreased insmad1/5morphants. Non-specific rabbit IgG was used as negative control (mean±s.d.,n=3,*P<0.05, Student’st-test). (h) ChIP assay was performed for theerk1(left) anderk2(right) promoter region in control embryos andsmad1/5morphants. DNA was immunoprecipitated with antibody against H3K9Ac or H3K27Ac. The acetylation level at H3K9 and H3K27 sites inerk1anderk2promoter region was increased insmad1/5morphants. Non-specific rabbit IgG was used as negative control (mean±s.d.,n=3,*P<0.05, Student’st-test). Figure 3: HDAC1 is recruited by Smad1/5 to regulate histone acetylation on the erk promoter. ( a ) The expression of runx1 at 24 hpf (left panels) and runx1 at 36 hpf (right panels) was decreased in the embryos treated with trichostatin A or valproic acid (VPA) and embryos injected with hdac1 MO (scale bar, 250 μm). ( b ) Quantitative RT–PCR analysis of erk1 and erk2 expression in the dissected trunk region of the embryos treated with TSA or VPA and embryos injected with hdac1 MO at 24 hpf (mean±s.d., n =3, *P <0.05, Student’s t -test). ( c ) Western blot showed that both pERK and total ERK protein levels were remarkably increased in the embryos treated with TSA or VPA and embryos injected with hdac1 MO at 24 hpf. ( d ) The diagram showed the Smad-binding sites in the erk1 and erk2 promoter region. The pair of arrows showed the primers designed for the ChIP assay. ( e , f ) ChIP-re-ChIP assay was performed for the erk1 ( e ) and erk2 ( f ) promoter region. Chromatin was precipitated with anti-pSmad1/5/8 or anti-HDAC1 antibody, and then re-precipitated with anti-HDAC1 or anti-pSmad1/5/8 antibody, respectively. Non-specific rabbit IgG was used as negative control (mean±s.d., n =3, *P <0.05, Student’s t -test). ( g ) ChIP assay was performed for the erk1 (left) and erk2 (right) promoter region in control embryos and smad1/5 morphants. DNA was immunoprecipitated with antibody against pSmad1/5/8 or HDAC1. The pSmad1/5/8 and HDAC1 enrichment was decreased in smad1/5 morphants. Non-specific rabbit IgG was used as negative control (mean±s.d., n =3, *P <0.05, Student’s t -test). ( h ) ChIP assay was performed for the erk1 (left) and erk2 (right) promoter region in control embryos and smad1/5 morphants. DNA was immunoprecipitated with antibody against H3K9Ac or H3K27Ac. The acetylation level at H3K9 and H3K27 sites in erk1 and erk2 promoter region was increased in smad1/5 morphants. Non-specific rabbit IgG was used as negative control (mean±s.d., n =3, *P <0.05, Student’s t -test). Full size image rVISTA (a database to search for evolutionarily conserved transcription factor binding sites) analysis indicated that there are several Smad-binding motifs in the upstream 5 kb region of erk1/2 promoter ( Fig. 3d ). To determine whether pSmad1/5 and HDAC1 can simultaneously bind to the endogenous erk1/2 promoter, we performed chromatin immunoprecipatation (ChIP)-re-ChIP assay in wild-type embryos using anti-pSmad1/5/8 antibody and anti-HDAC1 antibody, respectively. As expected, pSmad1/5 and HDAC1 co-existed in erk1 and erk2 promoter region ( Fig. 3e,f ). Furthermore, to test whether HDAC1 recruitment is dependent on pSmad1/5, ChIP assay was performed in smad1/5 and hdac1 morphants. It showed that both pSmad1/5/8 and HDAC1 enrichment in erk1/2 promoter region was decreased in smad1 or smad5 morphants ( Fig. 3g ), while pSmad1/5/8 enrichment in the hdac1 morphants was normal ( Supplementary Fig. 4c,d ). This indicated that Smad1 or Smad5 can recruit HDAC1 to the erk promoter region, and in the absence of Smad1 or Smad5, HDAC1 enrichment was significantly attenuated. It has been shown that there are histone acetylation peaks in erk1/2 promoter region (The University of California, Santa Cruz (UCSC) Genome Browser [33] ). We then quantified the level of H3K9- and H3K27 acetylation in smad1 and smad5 morphants and found that levels of both H3K9 and H3K27 acetylation were increased ( Fig. 3h ), suggesting that the increased H3K9 and H3K27 acetylation in the erk1/2 promoter after smad1/5 knockdown may facilitate their transcription due to the formation of more loose chromatin. To determine whether Smad1/5 directly regulates erk1/2 transcription, we performed reporter assay in HEK293T cells using the promoter constructs of erk1 and erk2 that contain conserved Smad-binding sites. Luciferase assays demonstrated that Smad1 and Smad5 negatively regulated erk1 and erk2 expression in a dose-dependent manner, especially with the cooperation of Hdac1 ( Supplementary Fig. 4e,f ). Taken together, Smad1 and Smad5 can recruit HDAC1 to the erk1/2 promoter region and then repress erk1/2 transcription through reducing histone acetylation (H3K9Ac and H3K27Ac). Endothelial-derived ERK mediates HSC development Since Smad1/5 inhibits ERK expression, we further investigate whether such inhibition is involved in regulating HSC development. erk2 MO was co-injected with smad1 or smad5 MO to rescue the HSC and vascular phenotype. Western blotting analysis showed that the augmentation of both ERK and pERK levels in smad1 and smad5 morphants was repressed by co-injection with erk2 MO ( Supplementary Fig. 5a ). Furthermore, WISH and qPCR results showed that the expression of HSC markers was restored by co-injection with erk2 MO ( Fig. 4a,b ). In the Tg( kdrl :mCherry/ cmyb :GFP) double-transgenic embryos, the decrease in number of kdrl + cmyb + cells was also restored by double knockdown of smads and erk2 ( Fig. 4c ). These results suggest that ERK mediates Smad1/5 regulation of HSC development. 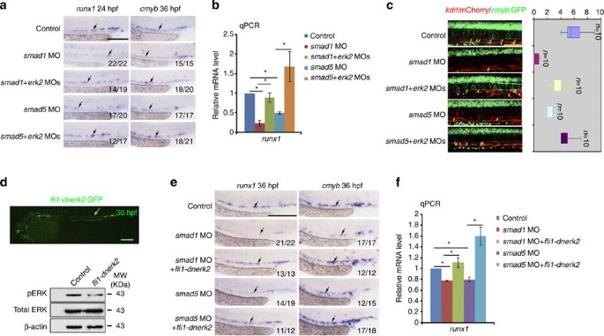Figure 4: Endothelial-derived ERK mediates Smad regulation of HSC development. (a)erk2MO partially rescued the expression ofrunx1at 36 hpf (left panels) andcmybat 36 hpf (right panels) insmad1orsmad5morphants (scale bar, 250 μm). (b) Quantitative RT–PCR analysis ofrunx1expression in the dissected trunk region of control embryos,smad1orsmad5morphants and rescued embryos by co-injection witherk2MO (mean±s.d.,n=3,*P<0.05, Student’st-test). (c) Confocal microscopy of Tg(kdrl:mCherry/cmyb:GFP) double transgenic line at 36 hpf in control embryos,smad1orsmad5morphants and rescued embryos by co-injection witherk2MO. The yellow arrows mark the haemogenic endothelial cells (scale bar, 100 μm). The right panel showed the statistics ofkdrl+cmyb+cell numbers in the trunk region (mean±s.d.,n=10). (d) The upper panel showed the GFP expression in endothelial cells in embryos injected with Fli1-ep-dnerk2:GFP at 30 hpf (scale bar, 250 μm). The lower panel showed that pERK protein level was downregulated at 24 hpf in embryos injected with Fli1-ep-dnerk2:GFP. (e) Fli1-ep-dnerk2:GFP partially rescued the expression ofrunx1at 36 hpf (left panel) andcmybat 36 hpf (right panels) insmad1orsmad5morphants (scale bar, 250 μm). (f) Quantitative RT–PCR analysis showed thatrunx1expression at 24 hpf was rescued by Fli1-ep-dnerk2:GFP insmad1orsmad5morphants (mean±s.d.,n=3,*P<0.05, Student’st-test). Figure 4: Endothelial-derived ERK mediates Smad regulation of HSC development. ( a ) erk2 MO partially rescued the expression of runx1 at 36 hpf (left panels) and cmyb at 36 hpf (right panels) in smad1 or smad5 morphants (scale bar, 250 μm). ( b ) Quantitative RT–PCR analysis of runx1 expression in the dissected trunk region of control embryos, smad1 or smad5 morphants and rescued embryos by co-injection with erk2 MO (mean±s.d., n =3, *P <0.05, Student’s t -test). ( c ) Confocal microscopy of Tg( kdrl: mCherry/ cmyb :GFP) double transgenic line at 36 hpf in control embryos, smad1 or smad5 morphants and rescued embryos by co-injection with erk2 MO. The yellow arrows mark the haemogenic endothelial cells (scale bar, 100 μm). The right panel showed the statistics of kdrl + cmyb + cell numbers in the trunk region (mean±s.d., n =10). ( d ) The upper panel showed the GFP expression in endothelial cells in embryos injected with Fli1-ep- dnerk2 :GFP at 30 hpf (scale bar, 250 μm). The lower panel showed that pERK protein level was downregulated at 24 hpf in embryos injected with Fli1-ep- dnerk2 :GFP. ( e ) Fli1-ep- dnerk2 :GFP partially rescued the expression of runx1 at 36 hpf (left panel) and cmyb at 36 hpf (right panels) in smad1 or smad5 morphants (scale bar, 250 μm). ( f ) Quantitative RT–PCR analysis showed that runx1 expression at 24 hpf was rescued by Fli1-ep- dnerk2 :GFP in smad1 or smad5 morphants (mean±s.d., n =3, *P <0.05, Student’s t -test). Full size image To determine whether ERK regulation of HSC development is conferred by endothelial cell-expressed ERK rather than ERK from other sources, a gateway construct was generated to express dominant-negative erk2 driven by Fli1 promoter ( fli1 - dnerk2 , Supplementary Fig. 5b ). This construct was generated by a K63R mutation, which blocks the phosphorylation of ERK at amino-acid residue 63 (ref. 34 ). GFP expression was detected in the vascular endothelial cells of embryos injected with fli1 - dnerk2 ( Fig. 4d ), confirming its specific expression in endothelial cells. Western blotting results showed that pERK level in the trunk region was decreased in fli1 - dnerk2 injected embryos, compared to the uninjected controls ( Fig. 4d ), which confirmed that fli1 - dnerk2 can attenuate endogenous ERK activity. fli1 - dnerk2 was then used to rescue runx1 expression in smad1/5 morphants. WISH and qPCR results showed that runx1 expression was rescued by ectopic vascular endothelial expression of dominant-negative form of erk2 ( Fig. 4e,f ). Taken together, ERK functions in the endothelial cells to restrict endothelium-derived HSC emergence. Over-activated ERK promotes arterial identity ERK pathway has been reported to function during the artery-vein specification and arterial morphogenesis [21] , [35] . The EHT process was inhibited in both erk2 MO and erk2 mRNA-injected embryos ( Supplementary Fig. 6a ). The phenotype in erk2 morphants may be caused by the impaired artery-vein specification, but how ERK over-activation inhibits HSC emergence is still unclear. Previous studies reported that HSCs emerged from the ventral wall of the dorsal aorta through losing the endothelial characters (such as endothelial cell identity or cell-cell adhesion) and acquiring haemogenic abilities sequentially [1] , [3] . We therefore asked whether overexpressed ERK could inhibit the haemogenic endothelial cell fate determination and the following EHT process through maintaining the aortic endothelial cell identity or enhancing the endothelial cell–cell adhesion. To test the hypothesis that overexpressed ERK could maintain the aortic endothelial cell identity, Tg( fli1a :EGFP) transgenic line was used. The endothelial cell expressed GFP was increased and the artery size was enlarged in smad1/5 morphants and erk2 mRNA-injected embryos ( Fig. 5a , left panel). Moreover, we counted the number of the aortic endothelial cell number using fli1a- nuclear-GFP transgenic lines Tg( fli1a :nGFP) ( Fig. 5a , middle panel). The transverse sectioning experiments showed that there were 4.2 cells on average in control embryos, while there were ~5 cells in smad1/5 morphants or erk2 mRNA-injected embryos, with statistical significance at a level of P <0.05 ( Fig. 5a , right panel). Expression of arterial markers dll4 , ephrinB2 and tbx20 was increased in both smad1/5 morphants and erk2 mRNA-injected embryos ( Fig. 5b ). Furthermore, the transverse sectioning post WISH showed that the expression of pan-endothelial cell marker cdh5 was also increased in the dorsal aorta in smad1/5 morphants and erk2 mRNA-injected embryos ( Fig. 5c ). qPCR results also agreed well with this observation, and showed that the increased expression of cdh5 in smad1/5 morphants could be rescued by erk2 MO co-injection ( Fig. 5d ). These results suggest that overexpressed erk in smad1/5 morphants enhanced the arterial endothelial cell identity. 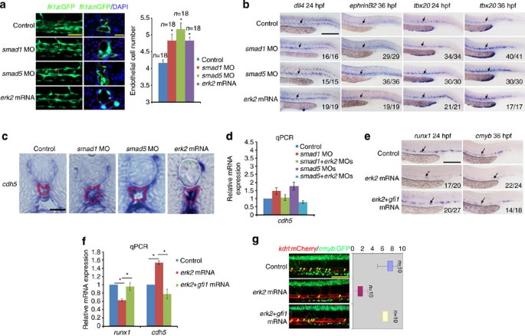Figure 5: Over-activated ERK inhibits the haemogenic endothelium determination by promoting the arterial endothelial cell identity. (a) The left panels showed the confocal microscopy of Tg(fli1a:EGFP) transgenic line at 36 hpf in embryos injected with control,smad1MO,smad5MO anderk2mRNA. Red lines mark the diameter of the dorsal aorta (scale bar, 50 μm). The middle panels showed the confocal microscopy of transverse section of injected Tg(fli1a:nGFP) embryos at 36 hpf. Red dotted lines mark dorsal aorta and green dotted lines mark posterior cardinal vein (scale bar, 20 μm). The right panel showed the statistics of endothelial cell numbers of the dorsal aorta wall on the transverse section in injected embryos (mean±s.d.,n=18,*P<0.05, Student’st-test). (b) The expression of arterial markerdll4,ephrinB2andtbx20in the dorsal aorta at 24 hpf and 36 hpf was increased in embryos injected withsmad1MO,smad5MO orerk2mRNA (scale bar, 250 μm). (c) Transverse sectioning post WISH showed that the expression of endothelial cell markercdh5at 24 hpf was increased in embryos injected withsmad1MO,smad5MO orerk2mRNA. The red dotted lines mark the dorsal aorta (scale bar, 50 μm). (d) Quantitative RT–PCR analysis showed that the increased expression ofcdh5insmad1orsmad5morphants was rescued by co-injection witherk2MO (mean±s.d., n=3,*P<0.05, Student’st-test). (e) The decreased expression ofrunx1at 24 hpf (left panels) andcmybat 36 hpf (right panels) inerk2overexpressed embryos was partially rescued by co-injection withgfi1mRNA (scale bar, 250 μm). (f) Quantitative RT–PCR analysis showed that the decreased expression ofrunx1at 24 hpf inerk2mRNA-injected embryos was rescued by co-injection withgfi1mRNA (mean±s.d.,n=3,*P<0.05, Student’st-test). (g) Confocal microscopy of Tg(kdrl:mCherry/cmyb:GFP) double transgenic embryos at 36 hpf co-injected withgfi1mRNA anderk2mRNA. The yellow arrows mark the haemogenic endothelial cells (scale bar, 100 μm). The right panel showed the statistics ofkdrl+cmyb+cell numbers in the trunk region (mean±s.d.,n=10). Figure 5: Over-activated ERK inhibits the haemogenic endothelium determination by promoting the arterial endothelial cell identity. ( a ) The left panels showed the confocal microscopy of Tg( fli1a :EGFP) transgenic line at 36 hpf in embryos injected with control, smad1 MO, smad5 MO and erk2 mRNA. Red lines mark the diameter of the dorsal aorta (scale bar, 50 μm). The middle panels showed the confocal microscopy of transverse section of injected Tg( fli1a :nGFP) embryos at 36 hpf. Red dotted lines mark dorsal aorta and green dotted lines mark posterior cardinal vein (scale bar, 20 μm). The right panel showed the statistics of endothelial cell numbers of the dorsal aorta wall on the transverse section in injected embryos (mean±s.d., n =18, *P <0.05, Student’s t -test). ( b ) The expression of arterial marker dll4 , ephrinB2 and tbx20 in the dorsal aorta at 24 hpf and 36 hpf was increased in embryos injected with smad1 MO, smad5 MO or erk2 mRNA (scale bar, 250 μm). ( c ) Transverse sectioning post WISH showed that the expression of endothelial cell marker cdh5 at 24 hpf was increased in embryos injected with smad1 MO, smad5 MO or erk2 mRNA. The red dotted lines mark the dorsal aorta (scale bar, 50 μm). ( d ) Quantitative RT–PCR analysis showed that the increased expression of cdh5 in smad1 or smad5 morphants was rescued by co-injection with erk2 MO (mean±s.d., n=3, *P <0.05, Student’s t -test). ( e ) The decreased expression of runx1 at 24 hpf (left panels) and cmyb at 36 hpf (right panels) in erk2 overexpressed embryos was partially rescued by co-injection with gfi1 mRNA (scale bar, 250 μm). ( f ) Quantitative RT–PCR analysis showed that the decreased expression of runx1 at 24 hpf in erk2 mRNA-injected embryos was rescued by co-injection with gfi1 mRNA (mean±s.d., n =3, *P <0.05, Student’s t -test). ( g ) Confocal microscopy of Tg( kdrl: mCherry/ cmyb :GFP) double transgenic embryos at 36 hpf co-injected with gfi1 mRNA and erk2 mRNA. The yellow arrows mark the haemogenic endothelial cells (scale bar, 100 μm). The right panel showed the statistics of kdrl + cmyb + cell numbers in the trunk region (mean±s.d., n =10). Full size image To further confirm the enhanced endothelial identity but decreased haemogenic activities of haemogenic endothelium and less EHT frequency, we analysed gfi1 expression. Gfi1 has been demonstrated to be critical for haemogenic endothelium by repressing endothelial markers [8] . Since gfi1 is expressed at the aorta–gonad–mesonephros (AGM) region [36] and is sufficient for HSC development ( Supplementary Fig. 6b ), we overexpressed gfi1 to rescue the increased endothelial identity in erk2- overexpressed embryos. The result showed that the decreased runx1 expression in erk2 -overexpressed embryos was partially rescued by gfi1 overexpression ( Fig. 5e,f ), and the number of kdrl + cmyb + cells was also restored ( Fig. 5g ). Furthermore, cdh5 expression was also rescued by gfi1 overexpression ( Fig. 5f ), indicating that gfi1 , as an endothelial repressor, could negatively mediate the ERK regulation of haemogenic endothelium determination. Over-activated ERK enhances the endothelial tight junction To test the hypothesis that overexpressed ERK could inhibit EHT process by enhancing the endothelial cell–cell adhesion, transmission electron microscopy (TEM) was performed. The results showed that the tight junction between arterial endothelial cells was strengthened in smad1/5 morphants or erk2 overexpressed embryos ( Fig. 6a ), which is most likely attributed to the increased ERK activity. To find out which adhesion molecule is involved in the ERK regulation of EHT process, we examined expression of a panel of the adhesion molecules including pecam , vcam1 , CD44a , lama4 and esam . We found that esam expression in the dorsal aorta was increased in smad1/5 morphants or erk2 -overexpressed embryos ( Fig. 6b ). Endothelial-specific adhesion molecule (ESAM) is a novel HSC-specific marker in mice [37] , [38] . Expression level of ESAM reflects the HSC transition status between quiescence and self-renewal [39] . It is also involved in the VEGF-triggered vascular permeability and Rho-mediated endothelial cell contacts [40] . Our results showed that the expression of esam was increased in these injected embryos ( Fig. 6b,c ), and such an increase in smad1/5 morphants could be rescued by erk2 MO co-injection ( Fig. 6c ). TEM imaging showed that the tight junction between vascular endothelial cells was disrupted in esam morphants but strengthened in the esam -overexpressed embryos ( Supplementary Fig. 6c ). Then, we asked whether esam was involved in the ERK regulation of EHT. WISH and qPCR results showed that the expression of runx1 and cmyb was increased in esam morphants but obviously decreased in esam -overexpressed embryos at 24 and 36 hpf ( Supplementary Fig. 6d,e ). We further employed esam MO to rescue the HSC defects caused by erk2 overexpression. The decreased expression of runx1 and cmyb in erk2 -overexpressed embryos was restored by co-injection with esam MO ( Fig. 6d,e ). Consistent with WISH results, the number of kdrl + cmyb + cells was also restored ( Fig. 6f ). However, the esam MO injection had no effect for the enhanced endothelial cell marker cdh5 in erk2 -overexpressed embryos ( Fig. 6e ). Strikingly, overexpression of gfi1 and knockdown of esam in erk2 -overexpressed embryos dramatically increased the expression of runx1 and cmyb ( Fig. 6d,e ) or the number of kdrl + cmyb + cells ( Fig. 6f ). 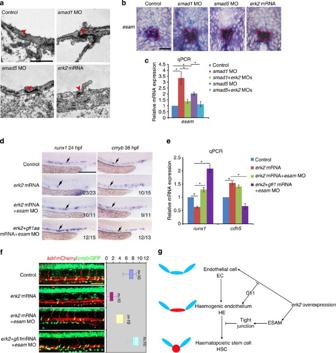Figure 6: Over-activated ERK inhibits the EHT process by enhancing the tight junction between endothelial cells. (a) Transverse TEM imaging showed that the endothelial cell junction (red arrowheads) was strengthened in embryos injected withsmad1MO,smad5MO orerk2mRNA (scale bar, 1 μm). (b) Transverse sectioning post WISH showed that the expression ofesamat 24 hpf was increased in embryos injected withsmad1MO,smad5MO orerk2mRNA. The red dotted lines mark the dorsal aorta (scale bar, 50 μm). (c) Quantitative RT–PCR analysis showed that the increased expression ofesaminsmad1orsmad5morphants was rescued by co-injection witherk2MO (mean±s.d., n=3,*P<0.05, Student’st-test). (d) The decreased expression ofrunx1at 24 hpf (left panels) andcmybat 36 hpf (right panels) inerk2-overexpressed embryos was partially rescued by co-injection withesamMO, and increased by co-injection with bothesamMO andgfi1mRNA (scale bar, 250 μm). (e) Quantitative RT–PCR analysis showed that the decreased expression ofrunx1at 24 hpf inerk2mRNA-injected embryos was rescued by co-injection withesamMO, and increased by co-injection with bothesamMO andgfi1mRNA (mean±s.d.,n=3,*P<0.05, Student’st-test). (f) Confocal microscopy of Tg(kdrl:mCherry/cmyb:GFP) double transgenic embryos at 36 hpf showed that co-injection withesamMO could rescue the reduced number ofkdrl+cmyb+cells inerk2mRNA-injected embryos. Co-injection with bothesamMO andgfi1mRNA dramatically increased the number ofkdrl+cmyb+cells inerk2-overexpressed embryos. The yellow arrows mark the haemogenic endothelial cells (scale bar, 100 μm). The right panel showed the statistics ofkdrl+cmyb+cell numbers in the trunk region (mean±s.d.,n=10). (g) Schematic model for the function of ERK2-Gfi1/Esam in regulating the different stages of EHT process. Figure 6: Over-activated ERK inhibits the EHT process by enhancing the tight junction between endothelial cells. ( a ) Transverse TEM imaging showed that the endothelial cell junction (red arrowheads) was strengthened in embryos injected with smad1 MO, smad5 MO or erk2 mRNA (scale bar, 1 μm). ( b ) Transverse sectioning post WISH showed that the expression of esam at 24 hpf was increased in embryos injected with smad1 MO, smad5 MO or erk2 mRNA. The red dotted lines mark the dorsal aorta (scale bar, 50 μm). ( c ) Quantitative RT–PCR analysis showed that the increased expression of esam in smad1 or smad5 morphants was rescued by co-injection with erk2 MO (mean±s.d., n=3, *P <0.05, Student’s t -test). ( d ) The decreased expression of runx1 at 24 hpf (left panels) and cmyb at 36 hpf (right panels) in erk2 -overexpressed embryos was partially rescued by co-injection with esam MO, and increased by co-injection with both esam MO and gfi1 mRNA (scale bar, 250 μm). ( e ) Quantitative RT–PCR analysis showed that the decreased expression of runx1 at 24 hpf in erk2 mRNA-injected embryos was rescued by co-injection with esam MO, and increased by co-injection with both esam MO and gfi1 mRNA (mean±s.d., n =3, *P <0.05, Student’s t -test). ( f ) Confocal microscopy of Tg( kdrl: mCherry/ cmyb :GFP) double transgenic embryos at 36 hpf showed that co-injection with esam MO could rescue the reduced number of kdrl + cmyb + cells in erk2 mRNA-injected embryos. Co-injection with both esam MO and gfi1 mRNA dramatically increased the number of kdrl + cmyb + cells in erk2 -overexpressed embryos. The yellow arrows mark the haemogenic endothelial cells (scale bar, 100 μm). The right panel showed the statistics of kdrl + cmyb + cell numbers in the trunk region (mean±s.d., n =10). ( g ) Schematic model for the function of ERK2-Gfi1/Esam in regulating the different stages of EHT process. Full size image Taken together, these data suggest that ERK overexpression inhibits the haemogenic endothelium formation through enhancing the endothelial cell identity, which could be repressed by GFI1, and then inhibits the EHT process through promoting the tight junction, which is mediated by ESAM ( Fig. 6g ). ERK inhibition by BMP–Smad1/5 is conserved in mouse AGM ERK, a central intracellular effector, plays pivotal roles in various cellular signalling across vertebrates and invertebrates [22] , [41] . We thus hypothesize that ERK inhibition by Smad5 in zebrafish HSCs might be also conserved in higher vertebrates, such as in mammals. To test this hypothesis, we took advantage of smad5 −/− knockout mice [42] , [43] . qPCR results showed that in the AGM region, the expression of erk1 and erk2 in smad5 −/− embryos was increased at embryonic day 8.5 (E8.5), E9.5 and E10.5 ( Fig. 7a , left and middle panel). In addition, expression of endothelial marker VE-cadherin and arterial markers ephrinB2 and dll4 was increased in the AGM region of smad5 −/− embryos at E10.5 ( Fig. 7a , right panel). Immunofluorescence showed that at E10, the stage when the earliest definitive HSCs are first derived from the AGM region of mouse embryos, the level of pSmad1/5/8 was remarkably reduced in the AGM region and the surrounding somites, whereas pERK and Dll4 were highly enriched in the dorsal aorta of smad5 −/− embryos ( Fig. 7b ). Runx1 expression in the AGM, which marks the definitive HSCs, was decreased in smad5 −/− embryos ( Fig. 7b ). These results were consistent with the elevated erk1/2 and pERK levels in blood vessels in zebrafish smad1 or smad 5 knockdown embryos, suggesting that this negative regulation of ERK signalling by Smad1/5 in definitive haematopoiesis is highly conserved from zebrafish to mouse. 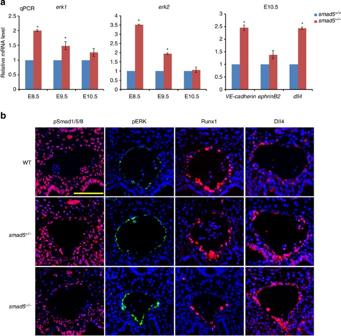Figure 7: Inhibition of ERK signalling by Smad5 is conserved in mice. (a) Quantitative RT–PCR analysis showed that the expression oferk1(left panel) anderk2(middle panel) was increased in the AGM region ofsmad5−/−mice at E8.5, E9.5 and E10.5. The expression ofVE-cadherin,ephrinB2anddll4(right panel) was increased in the AGM region ofsmad5−/−mice at E10.5 (mean±s.d.,n=3,*P<0.05, Student’st-test). (b) Immunofluorescence analysis showed the expression pattern of pSmad1/5/8, pERK, Runx1 and Dll4 in the AGM region of mouse embryos at E10. Note that the expression levels of pSmad1/5/8 and Runx1 were decreased, while that of pERK and Dll4 were increased in the AGM region ofsmad5−/−mice at E10 (scale bar, 250 μm). Figure 7: Inhibition of ERK signalling by Smad5 is conserved in mice. ( a ) Quantitative RT–PCR analysis showed that the expression of erk1 (left panel) and erk2 (middle panel) was increased in the AGM region of smad5 −/− mice at E8.5, E9.5 and E10.5. The expression of VE-cadherin , ephrinB2 and dll4 (right panel) was increased in the AGM region of smad5 −/− mice at E10.5 (mean±s.d., n =3, *P <0.05, Student’s t -test). ( b ) Immunofluorescence analysis showed the expression pattern of pSmad1/5/8, pERK, Runx1 and Dll4 in the AGM region of mouse embryos at E10. Note that the expression levels of pSmad1/5/8 and Runx1 were decreased, while that of pERK and Dll4 were increased in the AGM region of smad5 −/− mice at E10 (scale bar, 250 μm). Full size image To further confirm the conserved role of BMP-ERK in mouse haematopoiesis, endothelial cells, including haemogenic endothelial cells, from E10.5 AGM region were sorted and co-cultured with OP9-DL1 in the absence or presence of BMP specific inhibitor DMH1 (ref. 24) [24] ( Supplementary Fig. 7a ). The haematopoietic (cKit + CD45 + ) and haematopoietic-endothelial (cKit + CD31 + ) potential of the cultured cells was remarkably decreased when treated with DMH1, while the endothelial potential (cKit − CD31 + ) was increased ( Supplementary Fig. 7b ). For the CFU-C assay, the cultured cells were transferred to CFU-C media and cultured for 7 days. Numbers of representative colonies including BFU-E (burst-forming unit-erythroid), CFU-GM (colony-forming unit-granulocyte, macrophage) and mixed CFU-GEMM or CFU-Mix (colony-forming unit-granulocyte, erythroid, macrophage and megakaryocyte) were significantly reduced in DMH1-treated group ( Supplementary Fig. 7c ). To find out whether ERK expression was increased in this process, the abundance of total ERK and pERK was analysed by flow cytometry. Our results showed that the levels of both total ERK and pERK were increased in the DMH1-treated cells ( Supplementary Fig. 7d ). Taken together, these results confirmed that the BMP–Smad1/5 inhibition of ERK signalling is indispensable for haematopoiesis in mouse. In this study, we report the biphasic role of ERK signalling and a precise ERK signalling pulse to ensure a proper developmental sequence of HSCs in a stepwise manner in zebrafish and mouse embryos. As transcriptional factors, Smad1 and Smad5 transmit BMP signals into the nucleus and then regulate gene expression with the cooperation of transcriptional co-factors, including co-activators or co-repressors [44] . We found that Smad1/5 recruit HDAC1 to the erk1/2 promoter region to downregulate histone acetylation level (H3K9Ac, H3K27Ac), thereby decreasing erk1/2 transcription. Furthermore, we showed that over-activated ERK signalling in smad1/5 morphants can promote the arterial endothelial cell identity and strengthen the tight junction between endothelial cells through repressing gfi1 , which inhibits endothelial cell fate, and upregulating esam , a tight junction molecule, which ultimately leads to inhibition of the HSC initiation. Moreover, deficient ERK signals prior to artery-vein specification fail to establish the normal artery identity and thus affect the HSC production as well. With the input of BMP/Smad signals, the ERK activity may be kept at a balanced threshold level and maintains the homeostasis of HSCs during embryogenesis. Furthermore, this mechanism is conserved in mice as observed in embryos and AGM culture systems. This finding provides another additional layer of regulation of ERK signalling and specificity at the transcriptional level, other than the well-known Ras-Raf-MEK-ERK (MAPK) cascade. Previous studies showed that BMP/Smad pathway is indispensable for haematopoiesis. BMP is required to induce ventral mesoderm, which differentiates into haematopoietic and other mesoderm-derived tissues [45] . At the onset of definitive haematopoiesis, BMP pathway is required to trigger runx1 expression in the ventral wall of the dorsal aorta [15] , and also functions in the subaortic mesenchyme to promote HSC formation [46] . In this study, we found that BMP regulates the EHT process through direct inhibition of ERK expression via the cooperation between Smad1/5 and HDAC1. VEGF–ERK pathway is well known for its role in regulating artery specification [21] , [47] . Under normal conditions, VEGF–ERK signal is required to establish and/or maintain the artery-vein specification. It is previously demonstrated that functions of VEGF-ERK on HSC development depend on its role in artery-vein specification [19] . Our results were consistent with previous reports on this notion. In addition, we found that after artery-vein specification, ERK signalling pathway is not required for and conversely inhibits the HSC emergence by promoting the endothelial cell identity and tight junction. During vertebrate embryogenesis, the EHT process has been widely recognized as a major way of HSC production. Before EHT begins, a subset of endothelial cells in the ventral wall of dorsal aorta becomes haemogenic endothelial cells, which finally turn into HSCs via EHT. During this process, factors promoting arterial endothelial cell identity and the endothelial cell–cell adhesion should be repressed. Our study suggested that when the BMP pathway is inhibited, the endothelial-derived ERK signalling might be over-activated, which could inhibit the EHT process through promoting the aortic endothelial cell identity and strengthening cell–cell adhesion via ESAM. Under this condition, the haemogenic endothelial cells, if any, bind tightly to the surrounding endothelial cells and fail to bud off ( Supplementary Fig. 6a ); in addition, these cells have strong aortic endothelial cell identity ( Fig. 5 ), which is unfavourable for the transition process. BMP/Smad signal is essential to maintain ERK activity at a balanced level. Smad1/5 inhibits ERK expression at transcriptional level, which is mediated by recruiting HDAC1 to the erk promoter region. In smad1/5 -deficient embryos, ERK signalling was enhanced and that endothelial cell-specific dominant-negative ERK expression could rescue the HSC defects, further suggesting that the threshold level of ERK expression in endothelial cells is essential for sustaining haemogenic endothelium-derived HSC production. The relationship between BMP/Smad pathway and VEGF/ERK pathway has been examined in ESCs and early embryogenesis previously [28] , [48] , [49] . In Xenopus embryos, activated ERK can attenuate BMP signalling by phosphorylating the linker region of Smad1, which leads to the degradation of activated Smad1 to ensure the proper neural induction [48] , [49] . In mouse ESCs, BMP signalling pathway inhibits ERK activity through directly regulating Dusp9 expression to maintain the self-renewal of pluripotent ESC state [28] , [29] . However, there is no dusp9 homologue in zebrafish genome. Phylogenetic analysis showed that zebrafish dusp6 and dusp11 were orthologues of mouse dusp9 , but their expression was relatively unchanged in smad1/5 morphants. In this work, we showed that BMP inhibition of ERK signalling also exists in certain somatic stem cells (that is, HSCs), albeit unexpectedly, at the transcriptional level in zebrafish and mouse embryos. The transcriptional regulation of ERK expression is far from clear in the literature. ERK signalling is tightly regulated by the cooperation of transcription factors and epigenetic modification [5] , [22] , by which sustained or transient ERK activation thus exerts multiple effects in cell proliferation, differentiation and survival during development [41] . In our study, HDAC1 recruited by Smad1/5 was involved in the inhibition process of ERK expression at the transcriptional level during HSC development in vertebrate embryos. Such inhibition is important for HSC fate determination, which may provide a useful guide for the in vitro generation and expansion of HSCs from ESCs or iPSCs. For example, after generating the haemogenic endothelial cells from pluripotent stem cells in vitro , the BMP/Smad signal is required to promote the haematopoietic cell fate determination, while the VEGF/ERK pathway should be inhibited or kept at a very low level to suppress the endothelial cell identity of haemogenic endothelium, thereby facilitating the EHT process. So far, there is a serious lack of effective protocols to generate and expand HSCs in culture in vitro . Very recently, Pereira et al. [50] reported that a combination of four transcription factors can convert mouse fibroblasts into haemogenic endothelial intermediate that subsequently differentiates into HSPC-like cells. However, in vivo experiments including the lymphoid differentiation potential and long-term repopulation capacity have not been performed with these induced HSPC-like cells. Our study indicates that the fine-tuned balance between BMP and ERK signals must be tightly controlled to generate and maintain the HSCs in vivo . In summary, this work uncovers a novel cross-talk between BMP/Smad and ERK pathway during HSC emergence through EHT. BMP/Smad pathway directly inhibits ERK expression through recruiting HDAC1 to and inducing the de-acetylation of the erk promoter in haemogenic endothelial cells in vertebrate embryos. Such an inhibition thus maintains the equilibrium between the determination of haemogenic endothelial cell fate and the initiation of EHT process. The balanced control of ERK expression/activity by the cross-talk between BMP and ERK signalling, as part of an integrated regulatory network during HSC development, might also be extended to a broader context, in terms of cell fate decision, in general. This study provides new insights into the induction and maintenance of HSCs in vitro or ex vivo, which would pave a new way for designing novel methods for stem cell-based therapies. Animals Zebrafish embryos were obtained by natural spawning of adult Tubingen strain. Embryos were raised and maintained at 28.5 °C in fish water and staged as described previously [51] . Transgenic lines used in this study are summarized in Supplementary Table 1 . Embryos from these transgenic lines were staged to 10 hpf and subjected to heat shock at 42 °C for 30 min and then raised at 28.5 °C to the needed stage. The information of the chemical inhibitors used in this work is provided in Supplementary Table 2 . Smad5 knockout mice were obtained from the Institute of Biotechnology, Beijing, China. This study was approved by the Ethical Review Committee in the Institute of Zoology, Chinese Academy of Sciences, China. MOs and mRNA microinjection MOs were purchased from GeneTools, and prepared as 1 mM stock solutions using ddH2O. mRNAs were synthesized in vitro using the mMessage mMachine SP6 kit according to the manufacturer’s instruction (Ambion). For embryo injection, MOs and capped mRNA were injected into zebrafish embryos at the yolk/blastomere boundary at the one-cell stage. MO sequences were summarized in Supplementary Table 3 . WISH and transverse sections WISH for zebrafish embryos was performed as previously reported [52] with probes including runx1 , cmyb , erk1 , erk2 , dll4 , ephrinB2 , tbx20 , gfi1 , cdh5 and esam . Afterwards, the embryos were treated with 30% sucrose and washed three times with PBST. After being embedded in OCT complex (SAKURA), the embryos were sectioned using LEICA CM1900 Cryostats. Quantitative RT–PCR For zebrafish embryos, total RNAs were extracted from the trunk region (50 embryos pooled for each sample) at 24 hpf, and for mouse embryos, total RNAs were extracted from the trunk region of smad5 +/+ embryos at E8.5, E9.5 and E10.5 or smad5 +/+ and smad5 −/− embryos at E10.5 using TRNzol (Tiangen) and were reverse-transcribed using M-MLV Reverse Transcriptase (Promega). The obtained cDNAs were all diluted five times to be used as the templates for PCR amplification. The GoTaq qPCR Master Mix (Promega) was used for the quantitative RT–PCR analysis with the Bio-Rad CFX96 Real-Time PCR system. Data were represented as mean±s.d. and Student’s t -test was performed for comparison between control and experimental groups. All primers used for qPCR are presented in Supplementary Table 4 . ChIP and re-ChIP Chromatin immunoprecipitation (ChIP) analysis was performed with the trunk region of control embryos and smad1/5 morphants at 24 hpf; the eluted DNA precipitated by anti-pSmad1/5/8 (9511, Cell Signaling Technology), anti-HDAC1 (ab33278; Abcam), anti-H3K9Ac (07-352, Millipore) and anti-H3K27Ac (ab4729, Abcam) was evaluated by qPCR as described previously [52] . For re-ChIP, protein–DNA–bead complexes after initial overnight immunoprecipitation (anti-pSmad1/5/8 or anti-HDAC1) were washed three times with ChIP washing buffer, followed by double wash with 1 × TE buffer. Then, the washed immunoprecipitated protein–DNA complexes were incubated for 30 min at 37 °C in 75 μl of Re-ChIP elution buffer (1 × TE buffer, 2% SDS, 15 mM DTT, Protease inhibitor). After 600 g centrifugation, the supernatant was diluted 20 times (to a final volume of 1.5 ml) with ChIP dilution buffer, then proceeded with a second immunoprecipitation reaction with antibodies (anti-HDAC1 or anti-pSmad1/5/8). After extensive washing, the DNA was eluted using elution buffer (25 mM Tris-HCl, 10 mM EDTA, 0.5% SDS) and the eluted DNA was assayed by qPCR as described previously [53] . The primers specific to Smad-binding site within the upstream regulatory regions of erk1 and erk2 were designed. Rabbit purified IgG and non-specific primers were used as negative controls. Data were represented as mean±s.d. and Student’s t -test was performed for comparison between control and experimental groups. The primers and the expected product length are summarized in Supplementary Table 5 . Western blotting analysis Zebrafish embryos at 24 hpf were manually dechorionated, and the trunk region was homogenized with an 1-ml syringe and needle in cell lysis buffer (10 mM Tris-HCl, pH 8.0, 10 mM NaCl and 0.5% NP-40) containing protease inhibitor (Roche, catalogue number 04693116001) at 1 × concentration (one tablet in 2 ml redistilled water as 25 × concentration). Lysate was centrifuged at 12,000 g for 2 min at 4 °C and the resulting supernatant was loaded as protein samples. Western blotting was carried out as described previously [52] . The level of total ERK, pERK, β-Actin and Runx1 was detected by ECL method using the following antibodies: anti-ERK antibody (9102, Cell Signaling Technology, 1:1,000), anti-pERK antibody (9101, Cell Signalling Technology, 1:1,000), β-actin antibody (4967, Cell Signaling Technology, 1:2,000) and anti-Runx1 antibody (09-820, Upstate-Millipore, 1:100). Full scans of western blots are supplied in Supplementary Fig. 8 . Luciferase reporter assay The zebrafish erk1 and erk2 promoters were cloned and inserted into pGL3-luciferase vector. The zebrafish smad1 , smad5 and hdac1 full-length cDNAs were cloned into pCDNA3.1(+) vector. The pGL3-luciferase- erk1/erk2 promoter constructs and pCDNA3.1(+)- smad1/smad5/hdac1 constructs were transfected into HEK293T cells using Lipofectamine 2000 (Invitrogen). Luciferase activity was measured using the luciferase activity assay kit (Promega). Confocal microscopy Confocal images were acquired with a Zeiss LSM 510 META confocal laser microscope and three-dimensional (3D) projections were generated using Zeiss LSM software (Carl Zeiss Inc). Transmission electron microscopy Zebrafish embryos at 36 hpf, including control, erk2 or esam mRNA-injected embryos smad1/5 morphants, erk2 or esam morphants, were fixed in 2.5% glutaraldehyde in 0.1 M phosphate buffer solution (PBS, pH 7.0), and then postfixed in 1% osmium tetroxide for 2 h. All of the samples were dehydrated with a series of ethanol and then transferred to acetone. Finally, the samples were embedded in epoxy resin for ultrathin sectioning (70 nm). Sections were mounted on copper slot grids and stained with uranyl acetate and lead citrate. The images were taken using a JEM1400. Immunofluorescence smad5 +/+ , smad5 +/− and smad5 −/− embryos at E10 were fixed with 4% paraformaldehyde in phosphate-buffered saline (PBS) for 6 to 8 h at 4 °C. After fixation, the embryos were embedded in paraffin and cut in a microtome (Leica) to 5 μm and affixed onto the slides. H 2 O 2 solution (3%) was used to suppress endogenous peroxidase activity for 30 min at room temperature and antigen epitopes were retrieved with citrate buffer by microwave heating. Then, the precooled acetone was used for cellular membrane permeability. The slides were blocked with 10% goat serum for 1 h at room temperature and incubated with pSmad1/5/8 (9511, Cell Signaling Technology, 1:200), pERK (sc-7383, Santa Cruz, 1:250), Runx1 (ab92336, Abcam, 1:500) and Dll4 (ab7280, Abcam, 1:200) antibody diluted in 1% BSA overnight at 4 °C. After washing three times in PBST, the slides were incubated with anti-mouse-Ig-fluorescein or anti-rabbit-Ig-fluorescein for 1 h at room temperature. The sections were counterstained with DAPI and images were acquired by Nikon ECLIPSE 80i. FACS E10.5 AGMs (36–40 somite pairs) were dissociated by collagenase. Then, antibody staining was performed for 30 min on 4 °C using antibodies specific to CD31-PE (BD, 0.5 μg per test), CD41-FITC (eBioscience, 0.06 μg per test), CD45-APC (eBioscience, 0.125 μg per test), c-kit-APC (eBioscience, 0.06 μg per test) and TER119-PE-CY7 (eBioscience, 0.5 μg per test). The CD31 + CD41 − CD45 − TER119 − cells were sorted on a MoFlo XDP (BECKMAN COULTER). Single cells of the indicated numbers were cultured on mouse OP9-DL1 stromal cells and supplemented with haematopoietic cytokines (50 ng ml −1 SCF, 50 ng ml −1 IL3, 20 ng ml −1 FLT3 ligand. These cells were treated with DMSO and BMP inhibitor DMH1 respectively. After being cultured for 4 or 7 days, semi-adherent cells were carefully harvested to do CFC or flow cytometry. CFC assay Semi-adherent cells were carefully harvested and transferred to ultra-low attachment 24-well plates (COSTAR) and cultured in CFC media. The cells were incubated at 37 °C in 5% CO 2 with 100% humidity for 7 days, and the number of each type of colonies was counted according to morphology. The experiment was repeated in triplicate. Flow cytometric analysis Semi-adherent cells were carefully harvested. Then antibody staining was performed as described above, using antibodies specific to CD31-PE (BD), c-Kit-APC (eBioscience), CD45-PE (eBioscience). To evaluate the levels of ERK and p-ERK, cells were fixed, permeabilized and marked with total ERK (9102, Cell Signaling Technology, 1:50) or p-ERK antibody (9101, Cell Signaling Technology, 1:200). The primary antibodies were detected with Alexa Fluor 488-conjugated anti-rabbit IgG (Invitrogen). Statistical analysis All experiments were performed at least three times. Data are given as the mean±s.d. Student’s t -test was used for statistical comparisons. P <0.05 was considered significant. How to cite this article: Zhang, C. et al. Inhibition of endothelial ERK signalling by Smad1/5 is essential for haematopoietic stem cell emergence. Nat. Commun. 5:3431 doi: 10.1038/ncomms4431 (2014).